Programming adaptive control to evolve increased metabolite production The complexity inherent in biological systems challenges efforts to rationally engineer novel phenotypes, especially those not amenable to high-throughput screens and selections. In nature, increased mutation rates generate diversity in a population that can lead to the evolution of new phenotypes. Here we construct an adaptive control system that increases the mutation rate in order to generate diversity in the population, and decreases the mutation rate as the concentration of a target metabolite increases. This system is called feedback-regulated evolution of phenotype (FREP), and is implemented with a sensor to gauge the concentration of a metabolite and an actuator to alter the mutation rate. To evolve certain novel traits that have no known natural sensors, we develop a framework to assemble synthetic transcription factors using metabolic enzymes and construct four different sensors that recognize isopentenyl diphosphate in bacteria and yeast. We verify FREP by evolving increased tyrosine and isoprenoid production. Adaptation is a behaviour that allows cells to survive and thrive in constantly changing environmental conditions, and is characterized by rapid genetic change creating rare beneficial mutations [1] . The appearance of microbial strains with accelerated mutation rates accompany periods of adaptation in both natural and laboratory environments [2] , [3] , such as in the emergence of bacterial antibiotic resistance [4] . Models and experimental data of the adaptive process suggest that a ‘variable mutation rate’ strategy is one of the strategies used by nature to evolve traits, where a period of high mutation rate increases the genetic diversity of populations with low phenotypic diversity, and the mutation rate decreases with increased genetic diversity in the population [5] , [6] . Many mutagenesis strategies to generate diversity in the laboratory exist, but most industrially important phenotypes are not amenable to the high-throughput screens and selections required to isolate mutants exhibiting the desired traits [7] . Furthermore, directed evolution strategies that generate mutant libraries in vitro are limited by the ligation efficiency [8] , and those that use mutator strains with unregulated, high mutation rates to generate mutant libraries in vivo [9] suffer from the accumulation of deleterious mutations that eventually lead to cell death. Although adaptation has proven useful for evolving certain phenotypes, its application has been limited to traits that are directly tied to growth [10] , [11] , [12] . Therefore, a method capable of changing the mutation rate in vivo according to a particular phenotype, independent of whether it is linked to growth, could circumvent the constraints set by ligation inefficiencies, deleterious mutations, and assay availability. Here we create such a method by implementing the ‘variable mutation rate’ strategy to evolve increased metabolite production using an adaptive control system we call feedback-regulated evolution of phenotype (FREP). We demonstrate the utility FREP by evolving increased tyrosine and isoprenoid production. Feedback-regulated evolution of phenotype FREP consists of a two-module genetic circuit that dynamically controls the mutation rate of the genome ( M ) based on the concentration of a target metabolite ( L ) ( Fig. 1a ). The actuator module converts a transcriptional signal ( T ) into M , and the sensor module modifies T by converting L into a change in transcriptional signal (Δ T ). M affects L over time as mutations that increase the metabolite production accumulate in the genome, creating a feedback loop that causes M to decrease as L increases ( Fig. 1b ). FREP can successfully modify L by changing M , because the changes to the system are manifested through transcription, which occurs at a much faster timescale than the propagation of those changes through growth and cell division. The sensor is assembled from two components: a transcription factor (TF) that binds the target metabolite and a promoter regulated by the TF. Depending on the metabolite, FREP could evolve a phenotype at either the population or single-cell level. If the metabolite is diffusible across the cell membrane and the rate of diffusion >> dL/dt, then the effect of FREP is averaged across the entire population. However, if the metabolite is not diffusible across the cell membrane or its diffusion across the membrane is << dL/dt, then FREP acts on each individual cell separately. Here we demonstrate the application of FREP to the evolution at either the population or single-cell level, and use tyrosine as a membrane permeable and isopentenyl diphosphate (IPP) as a membrane-impermeable metabolite. 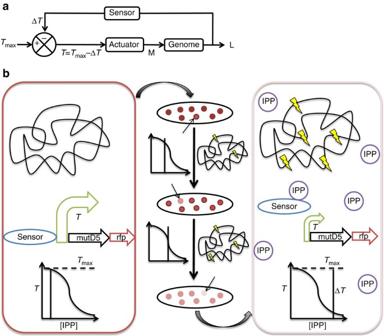Figure 1: FREP design. (a) FREP implementation of the variable mutation strategy using an adaptive control system. The sensor controls the change in transcriptional level (ΔT) in the system. The actuator converts the transcriptional level (T) into a mutation rate (M) that modifies the genome to produce the target phenotype gauged byL. AsLincreases, the sensor increases ΔT, which causes the actuator to decreaseM. (b) Evolution of increased IPP production using FREP. The sensor activates the promoter that controlsmutD5expression in the absence of the ligand IPP, and RFP acts as a reporter gene. MutD5 increases the mutation rate and mutations accumulate on the chromosome with each successive generation. Some of the mutations lead to increased IPP production, which decreases the ability of the sensor to activate expression ofmutD5andrfpin those cells. The mutations that increase IPP production are fixed into successive generations by passaging those cells with decreasedrfpexpression. Figure 1: FREP design. ( a ) FREP implementation of the variable mutation strategy using an adaptive control system. The sensor controls the change in transcriptional level (Δ T ) in the system. The actuator converts the transcriptional level ( T ) into a mutation rate ( M ) that modifies the genome to produce the target phenotype gauged by L . As L increases, the sensor increases Δ T , which causes the actuator to decrease M . ( b ) Evolution of increased IPP production using FREP. The sensor activates the promoter that controls mutD5 expression in the absence of the ligand IPP, and RFP acts as a reporter gene. MutD5 increases the mutation rate and mutations accumulate on the chromosome with each successive generation. Some of the mutations lead to increased IPP production, which decreases the ability of the sensor to activate expression of mutD5 and rfp in those cells. The mutations that increase IPP production are fixed into successive generations by passaging those cells with decreased rfp expression. Full size image FREP increases tyrosine production in E. coli We performed FREP to increase production of the industrially important amino-acid tyrosine [13] in Escherichia coli using the tyrosine-responsive TF TyrR [14] to regulate expression of the mutator mutD5 (ref. 15 ) ( Fig. 2 ). The mutD5 mutations are located in the mutD ( dnaQ ) gene that encodes the proofreading exonuclease of DNA polymerase III and leads to a reduction in mismatch repair. In this implementation, M should be high initially because the tyrosine concentration ( L ) is low, and M is reduced as beneficial mutations that increase tyrosine production appear. We modified TyrR and three TyrR-regulated promoters (P aroF , P aroL , P aroP ) to construct twenty different sensors, and screened their response to tyrosine in E. coli DJ106 and DJ166, two derivatives of BLR that produce different amounts of tyrosine. We monitored each sensor’s output with the fluorescent protein mCherry ( Supplementary Figs S1–S3 ). Sensor S aroF3 was the most sensitive to changes in tyrosine concentration, showing a 25% decrease in fluorescence from the lower to higher producing strain and a dynamic range of 0.44 RFU mM −1 per OD ( Fig. 3a ). 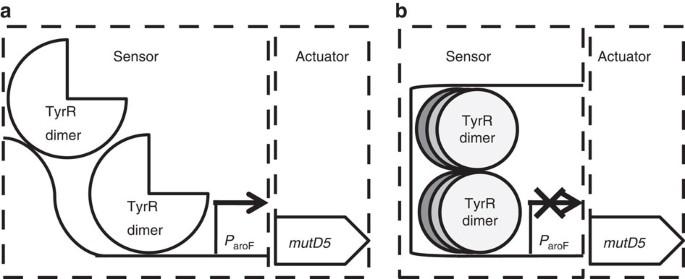Figure 2: FREP design to increase tyrosine production. (a) In one design, the sensor consists of TyrR and ParoF, and the actuator consists ofmutD5. TyrR dimers activate transcription from ParoFin the absence of tyrosine. (b) Tyrosine-bound TyrR form hexamers that dimerize to repress transcription from ParoF. Figure 2: FREP design to increase tyrosine production. ( a ) In one design, the sensor consists of TyrR and P aroF , and the actuator consists of mutD5 . TyrR dimers activate transcription from P aroF in the absence of tyrosine. ( b ) Tyrosine-bound TyrR form hexamers that dimerize to repress transcription from P aroF . 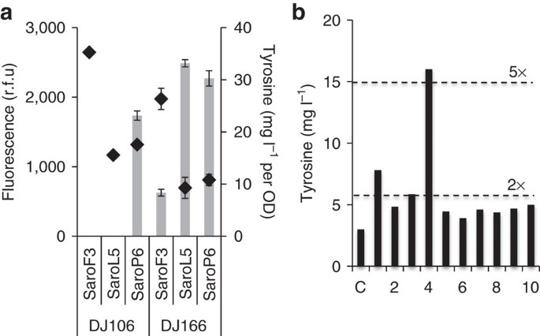Figure 3: FREP evolves increased tyrosine production. (a) Out of twenty sensors tested, the most sensitive sensors for each promoter (ParoF, ParoL, ParoP) are compared for sensitivity to changes in tyrosine concentrationin vivo. Bars represent tyrosine production and solid diamonds represent relative fluorescence units normalized to OD measured at 600 nm. DJ106 and DJ166 are variants ofE. coliBLR, and DJ166 produces more tyrosine than DJ106. The error bars represent s.d. Each data point represents the average of three replicates. (b) Tyrosine production from 10 mutants evolved with FREP showing the lowest fluorescence after 24 h. C is the control not evolved with FREP. Full size image Figure 3: FREP evolves increased tyrosine production. ( a ) Out of twenty sensors tested, the most sensitive sensors for each promoter (P aroF , P aroL , P aroP ) are compared for sensitivity to changes in tyrosine concentration in vivo . Bars represent tyrosine production and solid diamonds represent relative fluorescence units normalized to OD measured at 600 nm. DJ106 and DJ166 are variants of E. coli BLR, and DJ166 produces more tyrosine than DJ106. The error bars represent s.d. Each data point represents the average of three replicates. ( b ) Tyrosine production from 10 mutants evolved with FREP showing the lowest fluorescence after 24 h. C is the control not evolved with FREP. Full size image We tested FREP implemented with S aroF3 as the sensor and mutD5 as the actuator in E. coli DJ238, expressing mCherry bicistronically with mutD5 to monitor T and the relative mutator and metabolite levels in the cell. We reasoned that mCherry levels could decrease in response to either increased tyrosine production or mutations disrupting the sensor or mCherry expression. We isolated 10 colonies with the lowest fluorescence after 24 h and quantified tyrosine production to distinguish between the different scenarios. All 10 mutants demonstrated increased tyrosine production, and one exhibited greater than fivefold increase compared with the starting strain ( Fig. 3b ). Our observations indicate that raising M increased the diversity in the population to a level sufficient for mutants with increased L (tyrosine) to appear, and the sensor identified those mutants with increased metabolite production. A synthetic TF for IPP in E. coli To determine if FREP could evolve other traits, we implemented an adaptive control system to increase the production of isoprenoids, a class of compounds with a wide range of industrial applications, such as pharmaceuticals [16] and biofuels [17] . Natural TFs for these compounds have not been discovered yet, so we developed a framework to rationally assemble synthetic TFs that could be used to regulate evolution towards high isoprenoid-producing strains. Our strategy was to construct synthetic TFs reminiscent of natural TFs by taking advantage of their structural and functional modularity. The framework assembles synthetic TFs from three parts: Part1 is a metabolic enzyme that binds the target ligand, Part2 converts the binding signal into Δ T by regulating RNA polymerase binding to the target promoter, and Part3 joins Part1 and Part2 together ( Fig. 4a ). 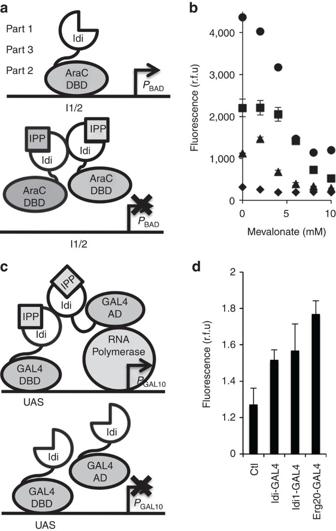Figure 4: Synthetic transcription factors respond to IPP. (a) A synthetic transcription factor (TF) consists of three parts: Part1 binds the target ligand, Part2 converts the binding signal into a change in RNA polymerase binding to the target promoter and Part3 is an amino-acid linker fusing Part1 and Part2 together. Here, a sensor with synthetic TF IA comprises Idi as Part1 and AraC’s DBD and linker as Part2 and Part3, respectively. One model for how IA regulates PBADis IA binds the DNA sequence I1I2, activating transcription from PBADin the absence of IPP (top), and IPP-bound IA dimerizes, preventing binding to I1I2and activation of PBAD(bottom). (b) Output of four sensors, each with a different TF, to changing IPP concentrations inE. coliHC175 monitored withmcherry. Solid diamonds represent AC, solid triangles IA32, solid squares IA and solid circles IA44. The error bars represent s.d. Each data point represents the average of three replicates. (c) A sensor for detecting IPP inS. cerevisiae. The synthetic TF consists of Idi as Part1, GAL4’s AD and DBD as Part2, and a 19-amino-acid linker as Part3. One model forPGAL10regulation is that Idi dimerizes when bound to IPP, bringing the upstream activation sequence (UAS)-bound GAL4 DBD in close enough proximity with the GAL4 AD to activate transcription (top). In the absence of Part1 dimerization, there is no transcription fromPGAL10(bottom). (d)PGAL10output from three sensors with synthetic TFs inS. cerevisiaeMO219 induced with galactose. The synthetic TFs consist of Idi, Idi1 or Erg20 as Part1 fused to GAL4’s AD and DBD. Ctl is the control without synthetic TFs. Output was monitored with the fluorescent protein yEcitrine and normalized to fluorescence in the absence of galactose. The error bars represent s.d. Each data point represents the average of three replicates. Figure 4: Synthetic transcription factors respond to IPP. ( a ) A synthetic transcription factor (TF) consists of three parts: Part1 binds the target ligand, Part2 converts the binding signal into a change in RNA polymerase binding to the target promoter and Part3 is an amino-acid linker fusing Part1 and Part2 together. Here, a sensor with synthetic TF IA comprises Idi as Part1 and AraC’s DBD and linker as Part2 and Part3, respectively. One model for how IA regulates P BAD is IA binds the DNA sequence I 1 I 2 , activating transcription from P BAD in the absence of IPP (top), and IPP-bound IA dimerizes, preventing binding to I 1 I 2 and activation of P BAD (bottom). ( b ) Output of four sensors, each with a different TF, to changing IPP concentrations in E. coli HC175 monitored with mcherry . Solid diamonds represent AC, solid triangles IA32, solid squares IA and solid circles IA44. The error bars represent s.d. Each data point represents the average of three replicates. ( c ) A sensor for detecting IPP in S. cerevisiae . The synthetic TF consists of Idi as Part1, GAL4’s AD and DBD as Part2, and a 19-amino-acid linker as Part3. One model for P GAL10 regulation is that Idi dimerizes when bound to IPP, bringing the upstream activation sequence (UAS)-bound GAL4 DBD in close enough proximity with the GAL4 AD to activate transcription (top). In the absence of Part1 dimerization, there is no transcription from P GAL10 (bottom). ( d ) P GAL10 output from three sensors with synthetic TFs in S. cerevisiae MO219 induced with galactose. The synthetic TFs consist of Idi, Idi1 or Erg20 as Part1 fused to GAL4’s AD and DBD. Ctl is the control without synthetic TFs. Output was monitored with the fluorescent protein yEcitrine and normalized to fluorescence in the absence of galactose. The error bars represent s.d. Each data point represents the average of three replicates. Full size image For example, AraC regulates expression of arabinose utilization genes from the arabinose-inducible araBAD promoter (P BAD ) by preferentially binding different DNA sequences in the presence and absence of arabinose [18] . AraC has a distinct amino-terminal, ligand-binding domain (LBD) and carboxy-terminal, DNA-binding domain (DBD), and changes its ability to activate or repress P BAD depending on whether the LBD has bound arabinose. We reasoned it should be possible to construct synthetic TFs for isoprenoids by replacing AraC’s LBD with metabolic enzymes that naturally bind isoprenoids. We engineered a synthetic E. coli TF (chimeric protein IA, Fig. 4a ) to respond to IPP, the central intermediate for all isoprenoid biosynthesis [19] , by fusing the AraC DBD (Part2) and linker (Part3) with IPP isomerase ( idi [20] ) (Part1). We chose Idi, because crystallographic data indicated that it dimerizes upon binding IPP [21] , suggesting that dimerization of Part1 could create at least two different conformational states for IA. We hypothesized that only one of the two states would activate transcription. A sensor consisting of IA and P BAD was tested by monitoring its output with mCherry in a modified strain of E. coli MG1655 able to convert mevalonate to IPP (HC175). A titration of mevalonate from 0–10 mM changed fluorescence by over threefold ( Fig. 4b ). There was no change in fluorescence when a synthetic TF consisting of only the AraC DBD and linker (AC) regulated P BAD . We also evaluated expression from the divergent araC promoter ( P c ) with cfp ( Table 1 ). Combined with the P BAD data, IA appears to regulate P BAD and P C nearly as tightly as AraC. Unlike AraC, IA represses P BAD in the presence of ligand. Furthermore, both half-sites I 1 and I 2 upstream of P BAD are necessary but interchangeable for IA regulation ( Supplementary Table S1 ). These observations indicate IA can regulate T from P BAD based on the concentration of L (IPP) with a fluorescent output of 518–2,202 r.f.u. per OD across a concentration range from 0–8 mM to provide a dynamic range of 210 r.f.u. mM −1 per OD, assuming all of the mevalonate was converted to IPP. Table 1 Fluorescence output from P BAD and P C . The promoters P BAD and P C were regulated by one of three TFs: AC, AraC, or IA. P BAD was monitored using RFP and P C with CFP. Full size table We purified IA to confirm it binds the I 1 and I 2 half-sites adjacent to P BAD in vitro . Gel electrophoresis mobility shift assay [22] experiments showed two bands when I 1 and I 1 I 2 were substrates and three bands when the substrate was the DNA sequence from P C to P BAD ( Supplementary Fig. S4 ). The additional band supports the observation that IA regulates both P BAD and P C , which have distinct binding sequences. The shifted DNA bands were less intense when IPP was added, indicating that IA’s affinity for the binding sequences decreases in the presence of IPP. We confirmed that IPP modulates IA DNA binding using fluorescence resonance energy transfer by splitting I 1 and I 1 I 2 into two DNA fragments each constituting half of the original sequence and tagged with either a fluorophore or quencher [23] . Only the presence of IA and both half-sequences induced a change in fluorescence ( Supplementary Fig. S5 ). Adding IPP decreased the change in fluorescence across all concentrations of IA tested ( Supplementary Fig. S6 ). Thus, both in vivo and in vitro data are consistent with IA regulation of transcription from P BAD according to changing IPP concentrations, and both I 1 and I 2 half-sites are necessary for this regulation. A synthetic TF for IPP in yeast To further evaluate our framework for assembling synthetic TFs, we constructed a synthetic TF for isoprenoids in Saccharomyces cerevisiae using the GAL4 protein, which regulates expression of GAL genes in response to galactose [24] . Similar to AraC, the functional domains of GAL4 are structurally distinct, consisting of an activator domain (AD) and DBD [25] . We reused Idi as Part1 and fused it to the GAL4 AD and DBD (Part2), reasoning that Idi dimerization should bring the AD and DBD in close enough proximity to activate transcription from a GAL promoter (for example, P GAL10 ). Part3 was a 19 amino-acid sequence having relatively high stability [26] . This sensor ( Fig. 4c ) was tested by monitoring its output with the fluorescent protein yEcitrine in S. cerevisiae MO219, a genetically modified strain that increases isoprenoid production when induced with galactose [27] . We observed a change in fluorescence greater than baseline after galactose induction ( Fig. 4d ). Two additional yeast TFs were constructed from yeast enzymes known to catalyse reactions with IPP as a substrate (Idi1 (ref. 28 ) and Erg20 (ref. 29 )) as Part1 in place of Idi, and both showed even greater changes in fluorescence following induction. Induction led to an almost twofold increase in sensor output in response to increased isoprenoid levels using the synthetic TF constructed with Erg20. Combined with IA, these GAL4-based TFs highlight the modularity of our framework in assembling synthetic TFs for constructing sensors, alleviating the need to rely on pre-existing biological components. FREP increases isoprenoid production in E. coli Next, we modified the E. coli IPP TF IA using error-prone PCR to create IPP sensors with different dynamic ranges and maximum transcription levels ( T max ). Out of the 60 variants screened ( Supplementary Fig. S7 ), IA32 (L39M, S127C) showed half the T max of IA and a dynamic range of 145 r.f.u. mM −1 per OD, whereas IA44 (R267H) showed twice the T max of IA and a dynamic range of 350 r.f.u./mM/OD ( Fig. 3c ). We implemented FREP using one of three synthetic TFs (AC, IA32 or IA44) as part of the sensor and the mutD5 actuator, and examined these constructs in E. coli MG1655 using Luria–Delbruck fluctuation analysis [30] . The fluctuation analysis data was analysed using the fluctuation analysis calculator web tool in order to calculate the mutation frequency and rate from a mutation assay that is based on the frequency of rifampicin resistance in the population. Thirty colonies for each implementation were tested for rifampicin resistance, an orthogonal phenotype that could be quantified quickly. In general, we observed more rifampicin-resistant mutants with higher mutator expression, and a strong correlation between relative mutator expression and mutation rate ( r =0.97) ( Supplementary Fig. S8 ). For example, IA32 and IA44 exhibited a fourfold difference in T max and a 2.4-fold difference in M . A negative control consisting of a sensor with IA44 and no actuator generated no rifampicin-resistant mutants. These results show that increasing Δ T decreases M , consistent with our design, and suggest that dynamically controlling mutator expression changes the mutation rate in the cell. Furthermore, the ability to adjust the dynamic range of the TF allows the range of metabolite concentration FREP can sense to be controlled. We performed FREP with IA44 to increase isoprenoid production in E. coli MG1655, and expressed mCherry bicistronically with the actuator to monitor changes in in vivo IPP concentration. Ten colonies with the lowest fluorescence after 24 h were made electrocompetent and transformed with a plasmid containing the lycopene synthase genes (pLyc). Lycopene measured from a random transformant for all 10 colonies was higher than the control without the actuator module. Six colonies had mutants producing on average 2,900 μg lycopene g −1 dry cell weight (p.p.m. ), a nearly threefold increase compared with the control that did not undergo FREP, which produced only 1,000 p.p.m. ( Supplementary Fig. S9 ). Repeating the experiment with a sensor employing AraC induced with arabinose as a negative control (AraC does not respond to IPP) generated no mutants producing more lycopene than the initial strain, illustrating the importance of the feedback loop and sensor to select mutants exhibiting increased metabolite production. Finally, we examined the ability of FREP to generate increased metabolite production in the context of a long-term experiment. We co-transformed pLyc with an IPP sensor and mutD5 actuator into E. coli MG1655, and monitored the evolution of IPP production using lycopene as a reporter over 432 h. We quantified lycopene production every 72 h from 10 random colonies and only passaged the isolate demonstrating the highest production levels. After 432 h, lycopene production increased to 6,800 p.p.m. using IA44, 4,700 p.p.m. using IA32, and only 400 p.p.m. using AraC ( Fig. 5a ). A negative FREP control implemented with IA44 without an actuator produced 0 p.p.m. For the strains evolved using FREP implemented with IA44 and an actuator, we purified pLyc from cells isolated from each time point. Transforming those plasmids into E. coli MG1655 did not lead to more lycopene production compared with the original plasmid ( Supplementary Fig. S10 ). This observation indicates that FREP generated mutations on the chromosome that are necessary for increased IPP production. No difference in growth rate was observed between the control and mutant strains. The absence of any changes in growth rate might be a result of our selection method. Cells were grown on plates prior to selection, and selection for high producers was done based on the intensity of the red colour of the colonies. Therefore, mutants with slower growth rates or slower production rates were selected against, and the mutants we propagated and analysed were those that grew and produced lycopene the fastest. It is possible that some of the slower growers might be higher producers, and we missed these mutants based on our selection criteria. 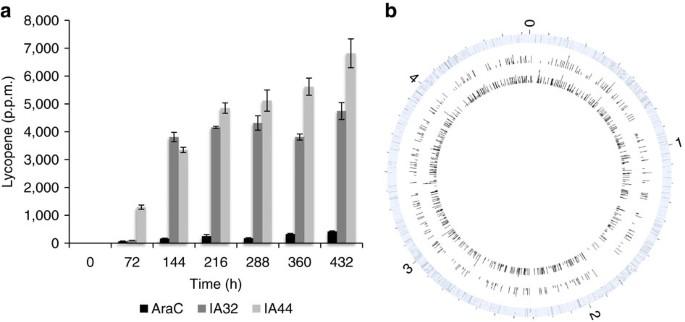Figure 5: FREP evolves increased IPP production. (a) Lycopene production sampled every 72 h over a 432-h period fromE. coliMG1655 expressing pLyc, an IPP sensor and an actuator. The transcription factors used in the sensor were AraC (black bars), IA32 (dark grey bars) or IA44 (light grey bars). Lycopene production is presented as p.p.m. (ug g−1dry cell weight). The sensor with AraC was induced with 10 mM arabinose. The error bars represent s.d. Each data point represents the average of three replicates. (b) The strains isolated at each 72-h timepoint for lycopene analysis were resequenced. The outer blue ring represents theE. coligenome, the middle blue ring represents the location of the nonsynonymous SNPs and the inner ring shows all of the SNPs. The height of the bars in the inner two rings illustrates the relative occurrence of each SNP, where a taller bar indicates that the SNP was identified in more of the strains isolated. Figure 5: FREP evolves increased IPP production. ( a ) Lycopene production sampled every 72 h over a 432-h period from E. coli MG1655 expressing pLyc, an IPP sensor and an actuator. The transcription factors used in the sensor were AraC (black bars), IA32 (dark grey bars) or IA44 (light grey bars). Lycopene production is presented as p.p.m. (ug g −1 dry cell weight). The sensor with AraC was induced with 10 mM arabinose. The error bars represent s.d. Each data point represents the average of three replicates. ( b ) The strains isolated at each 72-h timepoint for lycopene analysis were resequenced. The outer blue ring represents the E. coli genome, the middle blue ring represents the location of the nonsynonymous SNPs and the inner ring shows all of the SNPs. The height of the bars in the inner two rings illustrates the relative occurrence of each SNP, where a taller bar indicates that the SNP was identified in more of the strains isolated. Full size image We re-sequenced the strains isolated for high lycopene production as well as their parent strain. The parent strain matched the genome sequence of wild-type E. coli K12 MG1655 (GenBank: NC000913). The total number of SNPs and the number of non-synonymous SNPs increased with the amount of time FREP progressed until the final time point, where the number of SNPs remained the same and non-synonymous SNPs decreased. Between 0 and 360 h, the number of non-synonymous SNPs increased by 87, 250, 84, 4%, respectively. The decrease in the rate of accumulation of SNPs after 216 h confirms that the mutation rate decreased as the amount of IPP increased. The majority of the non-synonymous mutations is in the coding regions of the genome and is evenly distributed across the entire genome ( Fig. 5b ). Mutations in rrfD , rrfF , rrfG and ppiC were maintained in all of the strains collected throughout the 432 h of evolution. The rrf genes encode the 50S subunit of the ribosome, and mutations in these genes are in accordance with the previous efforts to modify the E. coli and S. cerevisiae transcription machineries [31] , [32] . These mutations suggest that modification to global mechanisms that affect the expression of multiple genes is an efficient mechanism to evolve new phenotypes. Related to the mechanism of translation, mutations were also found in infB , which is involved in translation initiation, rhlB and rne , which are involved in RNA catabolism. It is possible that some of the mutations accumulated might counter the deleterious effects of mutD5. Out of all of the genes that contain SNPs after undergoing FREP, only one gene, aceE , was previously identified to affect lycopene production [33] . These results illustrate the difficulty in predicting all of the genes involved in producing a particular phenotype, and how FREP enables a more complete exploration of the genomic search space to evolve a particular phenotype. We successfully designed and implemented an adaptive control process capable of implementing a variable mutation strategy and selecting for mutants that demonstrate increased production of a target metabolite. FREP is different from simulation and omics-based strategies, because it does not rely on preexisting knowledge about the genes, RNA, proteins and their interactions that govern the trait being engineered to decide what changes to make [33] , [34] . FREP is unique from other adaptive and metabolic evolution approaches [10] , [11] , [12] , because it monitors the phenotype being engineered using a sensor that can be linked to a fluorescent readout, so the phenotype does not need to be linked to growth. Furthermore, FREP hijacks the cell’s native mechanism for generating mutations and can be implemented in the absence of sophisticated recombination methods and automation equipment. Engineering the production of a particular metabolite is a complex, multi-dimensional problem with an extremely large but discrete search space that must account for many variables. This makes the global optimum extremely difficult to identify. Therefore, most methods to engineer microbial metabolism depend on current knowledge of metabolism and focus on engineering a very limited set of genes and proteins known to be associated with the production of the metabolite of interest. FREP takes a novel approach that resembles the simulated annealing method of optimization based on the Metropolis Hastings algorithm for optimization of nonlinear systems. The large search space associated with optimizing metabolism makes direct sampling extremely difficult due to the practical limitations in generating that search space. Therefore, FREP generates a random library that attempts to represent that search space and tries to identify a good approximation of the global optimum in a fixed amount of time by changing the mutation rate. When the mutation rate is high, the probability that a new genome is fixed into the population is low. However, the mutation rate decreases as the concentration of the target metabolite increases, and the probability that a new genome is fixed into the population increases as the mutation rate decreases. The allowance for the mutation rate to increase rather than always decrease prevents FREP from getting trapped in a local optimum. We demonstrated the application of FREP by evolving E. coli to increase tyrosine and IPP production, and isolating the evolved strains by monitoring the actuator level with a fluorescent protein. We confirmed that FREP was able to evolve increased production of metabolites that are either permeable or impermeable to the cell membrane. Metabolites that are membrane impermeable appear to be easier to evolve using FREP than those that are permeable, as exemplified by the fact that two out of ten tyrosine mutants and six out of ten IPP mutants showed a more than twofold increase in production. Once the level of a target trait saturates using a particular TF, its dynamic range could be altered to enable further increases in the level of the trait using FREP. Although the final population evolved using FREP could be heterogeneous with slight variations in production, the same sensor could be used to identify those individuals with the highest production. For example, by transforming the population of mutants with a construct that contains the sensor and not the mutator, the concentration of the metabolite can be translated into a fluorescence signal that can be sorted using FACS in order to identify the highest producing individual. Nevertheless, selecting the mutants using the sensor would still be superior to sorting them using FACS. Additionally, we presented a framework to rationally construct synthetic TFs using metabolic enzymes that enable the development of orthogonal sensors less likely to interact with existing cellular networks without being limited to the molecular recognition properties and control functions of naturally occurring TFs. Oligonucleotides and DNA sequencing All oligonucleotides were obtained from Integrated DNA Technologies and are presented in Supplementary Table S2 . The function of each pair of oligonucleotides used to construct the plasmids in this study is described in Supplementary Table S3 . DNA sequencing was performed by Quintara Biosciences. Strains and plasmids availability Strains, plasmids and plasmid sequences (in Genbank format) are deposited in the private instance of the JBEI registry and will be moved to the public instance ( http://www.public-registry.jbei.org ) after publication. Strains and plasmids are available from Addgene ( http://www.addgene.org ), and listed in Supplementary Table S4 . Strains We cloned the kanamycin cassette from pKD4 into pMevB [35] to construct pMevB–Kan using the primers Kan-F and Kan-R. We engineered EcHC175 by amplifying mk , pmk and pmd of the mevalonate operon with the kanamycin cassette from pMevB–Kan with the primers IdiKO-F and IdiKO-R, and knocking out idi in E. coli MG1655 with the PCR product according to Datsenko & Wanner [36] . E. coli DJ106, DJ166 and DJ238 were gifts from Dr. Darmawi Juminaga. S. cerevisiae MO219 was a gift from Dr. Mario Ouellet. Genes and promoter sequences amplified from the E. coli chromosome were from MG1655. Genes amplified from the S. cerevisiae chromosome were from BY4742. Construction of pLyc We cut crtE , crtI and crtB from pT-LYCm4 (gift from Dr. Adrienne McKee) using the restriction enzymes SpeI and HindIII. The cut fragment was gel purified and ligated into pBAD18-Cm using T4 DNA ligase (Fermentas) in order to construct pLyc. The ligation product was transformed into E. coli DH10B using electroporation. Construction of plasmids containing E. coli IPP sensors pCtl-RFP-S AraC (S AraC : sensor containing AraC) was constructed by removing HindIII from pBAD24 using QuickChange PCR, cloning in the DNA sequence from araC to P BAD from pBAD24M-gfp [37] using ClaI and EcoRI, cloning in mutD amplified from E. coli , and cloning in mCherry 3′ of the araBAD promoter, P BAD . The chimeric protein IA was constructed by fusing idi to the C-terminus of araC using SOEing PCR. idi was amplified from E. coli , and the linker and C-terminus of araC were amplified from pBAD24. These two PCR products were templates for SOEing PCR to amplify the chimeric protein. We cloned IA into pCtl-RFP-S AraC by replacing AraC to make pCtl-RFP-S IA . Mutants of IA were generated using the GeneMorph II Random Mutagenesis Kit (Agilent Technologies) according to the manufacturer’s instructions. We cloned the IA mutants into pCtl-RFP-S IA , transformed the constructs into EcHC175, and screened for changes in RFP expression relative to IA in the presence (10 mM) and absence (0 mM) of mevalonate with 0.1 mM isopropyl β- D -1-thiogalactopyranoside (Sigma-Aldrich). RFP was measured using a Spectramax M2 (Molecular Devices) exciting at 587 nm and measuring emission at 610 nm. We isolated two mutants: IA32 and IA44. pCtl-RFP-S AC was constructed by amplifying the C-terminal domain of AraC, and cloning into pCtl-RFP-S AraC . pCtl-RFP-S IA44 was digested with ClaI and KpnI, and the fragment containing IA44 to mutD was cloned into pBAD24 to construct pCtl-S IA44 . Construction of plasmids containing mutD5 mutator module The mutator mutD5 was a gift from Dr. Adrienne McKee and cloned into pCtl-S IA44 , pCtl-RFP-S AraC , pCtl-RFP-S IA44 , and pCtl-RFP-S aroF3 using the primers MutD-F and MutD-R to make pMut-S IA44 , pMut-RFP-S AraC , pMut-RFP-S IA44 , and pMut-RFP-S aroF3 . pMut-S AC , pMut-S AraC , pMut-S IA32 were constructed by cutting the TF from pCtl-RFP-S AC , pCtl-RFP-S AraC , pCtl-RFP-S IA32 using ClaI and HindIII, and cloning the fragments into pMut-S IA44 . Characterization of E. coli IPP sensor modules We measured expression of RFP from P BAD controlled by one of the TFs (AraC, AC, IA, IA32 or IA44) by transforming pCtl-RFP-S (S designates a sensor with one of the TFs) into EcHC175 and plating on LB agar plates with ampicillin and kanamycin. We picked three clones from each plate, grew each clone in LB medium with antibiotics overnight and inoculated each culture into fresh EZ Rich Defined Medium (Teknova) with antibiotics to an initial Abs 600 of 0.05 the following day. Each fresh culture was grown for 3 h at 37 °C, induced with isopropyl β- D -1-thiogalactopyranoside (0.1 mM) and mevalonate (0–10 mM) (or 0–10 mM arabinose for AraC), and grown for an additional 17 h at 37 °C. We measured RFP fluorescence exciting at 495 nm and measuring emission at 520 nm, and Abs 600 using a Spectramax M2. To determine IA’s binding sequence upstream of P BAD , we amplified I 1 I 1 using the primer I1I1-F, I 2 I 1 using the primer I2I1-F or I 2 I 2 using the primer I2I2-F, all paired with AraReg-R and using pCtl-RFP-S IA as template. The PCR products were cloned into pCtl-RFP-S IA to replace the I 1 I 2 sequence to make pCtl-RFP-S IA -I 1 I 1 , pCtl-RFP-S IA -I 2 I 1 and pCtl-RFP-S IA -I 2 I 1 . RFP expression from the modified binding sequences was determined as described above. We amplified CFP using the primers CFP-F and CFP-R, and inserted it 3′ of the TF expressed 3′ of P C into pCtl-RFP-S AC , pCtl-RFP-S AraC , and pCtl-RFP-S IA to make pCtl-CFP-RFP-S AC , pCtl-CFP-RFP-S AraC , and pCtl-CFP-RFP- S IA . RFP and CFP expression from these constructs were determined as indicated above, and CFP fluorescence was measured using a Spectramax M2 exciting at 433 nm and measuring emission at 475 nm. Construction of plasmids containing tyrosine sensor modules We replaced P C with CP20 (ref. 38 ) in pCtl-RFP- S AraC and cloned in tyrR amplified from E. coli to construct pCtl-RFP-TyrR. pCtl-RFP-S aroF0 was constructed by amplifying the promoter region of aroF from E. coli and cloning the PCR product into pCtl-RFP-TyrR to replace P BAD . pCtl-RFP-S aroF1 was constructed by mutating TyrR to make TyrR E274Q [39] and cloning the PCR product into pCtl-RFP-S aroF0 . pCtl-RFP-S aroF2 was constructed by mutating TyrR to make TyrR N316K [40] , and cloning the PCR product into pCtl-RFP-S aroF0 . pCtl-RFP-S aroF3 was constructed by incorporating the N316K mutation into TyrR E274Q and cloning the PCR product into pCtl-RFP-S aroF0 . The N-terminus of TyrR was also truncated to different lengths to generate TyrR Δ43, TyrR Δ93, and TyrR Δ187 (ref. 41 ) to make pCtl-RFP-S aroF4 , pCtl-RFP-S aroF5 and pCtl-RFP-S aroF6 . pCtl-RFP-S aroL0 was constructed by replacing P BAD with the promoter region of aroL from E. coli and cloning the PCR product into pCtl-RFP-TyrR. TyrR from pCtl-RFP-S aroF1 , pCtl-RFP-S aroF2 and pCtl-RFP-S aroF3 were amplified and cloned into pCtl-RFP-S aroL0 to construct pCtl-RFP-S aroL1 , pCtl-RFP-S aroL2 and pCtl-RFP-S aroL3 , respectively. The TyrR boxes 1, 2, 3 of the promoter P aroL were also modified to tune TyrR regulation of the promoter [42] . pCtl-RFP-S aroL4 was constructed by modifying the sequences of box 1 and 2 of P aroL in pCtl-RFP-S aroL0 . pCtl-RFP-S aroL5 was constructed by modifying the box 3 sequence of P aroL in pCtl-RFP-S aroL0 . pCtl-RFP-S aroP0 was constructed by replacing P BAD with the promoter region of aroP from E. coli and cloning the PCR product into pCtl-RFP–TyrR. TyrR from pCtl-RFP-S aroF1 , pCtl-RFP-S aroF2 and pCtl-RFP-S aroF3 were amplified and cloned into pCtl-RFP-S aroP0 to construct pCtl-RFP-S aroP1 , pCtl-RFP-S aroP2 and pCtl-RFP-S aroP3 , respectively. pCtl-RFP-S aroP4 was constructed by modifying the P 2 sequence of P aroP to make P 2up [43] in pCtl-RFP-S aroP0 . pCtl-RFP-S aroP5 and pCtl-RFP-S aroP6 were constructed by amplifying TyrRΔ43 and TyrRΔ93 from pCtl-RFP-S aroF4 and pCtl-RFP-S aroF5 , respectively and cloning the PCR products into pCtl-RFP-S aroP4 . Characterization of tyrosine sensor modules Plasmids containing each of the 20 tyrosine sensors described above were transformed into E. coli DJ106 and DJ166, and plated on LB agar with ampicillin. Clones were grown overnight in LB medium with ampicillin, inoculated into EZ Rich Defined Medium the next day to an initial Abs 600 of 0.05, and tyrosine production was quantified after 20 h. RFP fluorescence and Abs 600 were measured as described earlier. The experiment was repeated in triplicate for S aroF3 , S aroL5 and S aroP6 . Yeast synthetic TFs and IPP sensor modules The TEF promoter was amplified and cloned into pESC-Ura to make pESC-P TEF . yEcitrine was amplified and cloned into pESC-P TEF behind P gal10 to make pESC-YFP-P TEF . The cyc1 terminator and TEF promoter were fused using SOEing PCR to make the PCR product P TEF2 . The activator (AD) and DNA-binding domains (DBD) of gal4 were amplified from S. cerevisiae and the PCR products were fused 5′ of E. coli idi , S. cerevisiae idi1 or S. cerevisiae erg20 using SOEing PCR. Each AD/DBD pair of fusion constructs was cloned into pESC-YFP-P TEF behind P TEF and separated by P TEF2 to make pESC-YFP-S Idi-GAL4 , pESC-YFP-S Idi1-GAL4 , and pESC-YFP- S Erg20-GAL4 . Characterization of yeast IPP sensor modules pESC-YFP-P TEF , pESC-YFP-S Idi-GAL4 , pESC-YFP-S Idi1-GAL4 and pESC-YFP- S Erg20-GAL4 were transformed into ScMO219 using electroporation, plated on synthetic defined (s.d.) agar without uracil and with 2% glucose, and grown at 30 °C for 3 days. s.d. medium was composed of 1 × CSM without the appropriate amino acids (Sunrise Science Products) and 1 × Difco Yeast Nitrogen Base without amino acids (BD), prepared according to the manufacturers’ instructions. Three clones from each plate were grown overnight in s.d. medium without uracil and with 2% glucose, inoculated into fresh medium without uracil and with 1.8% galactose and 0.2% glucose the following day to an initial Abs 600 of 0.05, and grown for 3 days at 30 °C. YFP fluorescence was measured using a Spectramax M2 (Molecular Devices) exciting at 516 nm and measuring emission at 529 nm and normalized to OD measured at 600 nm. Genbank accession numbers: Sequences of E. coli evolved with FREP for increased IPP production have been deposited in the NCBI Sequence Read Archive and are available through GenBank. The accession numbers for the sequences of the samples at the time points 0, 72, 144, 216, 288, 360 and 432 h are SRR956947 , SRR957648 , SRR958168 , SRR958194 , SRR 958276 , SRR958416 and SRR958812 , respectively. How to cite this article: Chou, H. H. & Keasling, J. D. Programming adaptive control to evolve increased metabolite production. Nat. Commun. 4:2595 doi: 10.1038/ncomms3595 (2013).